Fluorinated MOF platform for selective removal and sensing of SO2from flue gas and air Conventional SO 2 scrubbing agents, namely calcium oxide and zeolites, are often used to remove SO 2 using a strong or irreversible adsorption-based process. However, adsorbents capable of sensing and selectively capturing this toxic molecule in a reversible manner, with in-depth understanding of structure–property relationships, have been rarely explored. Here we report the selective removal and sensing of SO 2 using recently unveiled fluorinated metal–organic frameworks (MOFs). Mixed gas adsorption experiments were performed at low concentrations ranging from 250 p.p.m. to 7% of SO 2 . Direct mixed gas column breakthrough and/or column desorption experiments revealed an unprecedented SO 2 affinity for KAUST-7 (NbOFFIVE-1-Ni) and KAUST-8 (AlFFIVE-1-Ni) MOFs. Furthermore, MOF-coated quartz crystal microbalance transducers were used to develop sensors with the ability to detect SO 2 at low concentrations ranging from 25 to 500 p.p.m. Global warming and other environmental/ecological issues have forced our society to adopt stringent rules for industrial waste and be on the lookout for ways to improve indoor and outdoor air quality, including in industrial sites. One major form of industrial waste with an adverse effect on the environment is flue gas. Flue gas generated by large industries and power plants resulting from burning fossil fuel contains CO 2 (at a low percent concentration), SO 2 (500–2000 p.p.m. ), NO 2 (few p.p.m. ), water vapor, and nitrogen (as the dominant gas) [1] . Although the concentration of SO 2 in flue gas feed is low, it could be poisonous for most liquid- or/and solid-state-based CO 2 separating agents. Therefore, the removal of SO 2 from flue gas is of prime importance [2] . Current SO 2 removal technology involves the irreversible acid–base reaction of SO 2 with CaO to form CaSO 3 [3] . The main drawback of this technology is its relatively low removal efficiency (< 90%) associated with an almost impossible regeneration step due to its extremely energy-intensive cost. Therefore, cyclable physical sorption technology is perceived as an effective alternative approach. Hence, identification of an adsorbent that can efficiently capture SO 2 , particularly at low concentration (< 500 p.p.m. ), is crucial. When SO 2 is not controlled and is emitted into the atmosphere, it has adverse effects on the environment, such as acid rain, and must be monitored [4] , [5] . Therefore, it is necessary to find efficient solutions to sense SO 2 at p.p.m. level (above 25 p.p.m.) in both dry and humid conditions. Recently, there have been considerable efforts in developing SO 2 sensing devices based on metal oxides (such as SnO 2 , WO 3 , and TiO 2 ) due to their excellent sensitivity, selectivity, response time, and recovery time [6] , [7] , [8] , [9] , [10] . However, most of the semiconductor-based SO 2 sensors were reported to require high temperatures (200–600 °C), leading to high levels of power consumption [11] , [12] , [13] , [14] , [15] . There is therefore a need for gas sensors that operate at room temperature (RT) [16] , [17] , [18] , which would be an important parameter and invaluable milestone for developing alternate materials suitable for detecting SO 2 . Metal–organic frameworks (MOFs), one of the most recent classes of porous materials, have attracted immense interest due to their potential to address many enduring challenges pertaining to various key applications [19] , [20] , [21] such as separation, storage, catalysis, and sensing [22] , [23] , [24] . Although many of these MOFs possess good-to-excellent chemical stability (which is a prerequisite for practical industrial applications) [25] , [26] , there are only a few examples of SO 2 adsorption on MOFs, mainly due to its corrosive nature [27] , [28] , [29] , [30] , [31] , [32] , [33] , [34] , [35] , [36] . Many of these reported MOFs adsorb SO 2 irreversibly or undergo phase transformations and they are not suitable for SO 2 –structural-adsorption-sensing relationships studies; only a handful of MOFs are proven for cyclic stability and SO 2 capture at flue gas concentration [27] , [28] , [29] , [30] . In addition, designing a sensor device for reversible SO 2 sensing at p.p.m. level and in the presence of atmospheric moisture is still an ongoing challenge. Here we report the use of isostructural fluorinated MOFs for (i) selective removal of SO 2 from synthetic flue gas and (ii) sensing of SO 2 [37] , [38] using a quartz crystal microbalance (QCM) as a transducer [18] , [39] , [40] , [41] , as the coating of MOFs on the QCM electrodes can detect the change in mass of sub-nanograms upon adsorption or desorption of molecules by the MOF layer [42] , [43] . We unveiled an unprecedented concurrent removal of SO 2 /CO 2 from synthetic flue gas and remarkable detection capability in p.p.m. level of SO 2 concentration in both dry and humid conditions. SO 2 removal from flue gas Recently, our exploration of fluorinated MOF platforms, namely KAUST-7 ([Ni(NbOF 5 )(pyrazine) 2 ] · 2H 2 O, apparent surface area 280 m 2 g −1 , estimated pore volume 0.095 cm 3 g −1 ) and KAUST-8 ([Ni(AlF 5 (OH 2 )) (pyrazine) 2 ] · 2H 2 O, apparent surface area 258 m 2 g −1 , estimated pore volume 0.102 cm 3 g −1 ), resulted in many desirable properties that include direct air capture [44] , propane-propylene separation [45] , gas/vapor dehydration [46] , and acid gas (H 2 S, CO 2 ) removal [47] . Although both of the MOFs are isostructural, the subtle differences in their chemical compositions, pillared by the inorganic moiety (NbOF 5 ) 2− instead of (AlF 5 (OH 2 )) 2− , allowed the modulation of their properties by varying the content and intermolecular spacing of pending fluoride groups realized via different tilts of pyrazine molecules (Fig. 1 ). Inspired by the excellent stability and the modular nature of these MOF materials [44] , [45] , [46] , we investigated their SO 2 removal and sensing in synthetic flue gas and air, respectively. Fig. 1 Synthesis and crystal structure of KAUST-7 and KAUST-8. a [Ni(pyrazine) 2 ] 2+ square grid resulting from the connection of Ni 2+ cations and pyrazine molecules. b Crystal structure of KAUST-8 resulting from the pillaring of [Ni(pyrazine) 2 ] 2+ square grid with (AlF 5 (OH 2 )) 2− pillar. c Crystal structure of KAUST-7 resulting from the pillaring of [Ni(pyrazine) 2 ] 2+ square grid with (NbOF 5 ) 2− pillar Full size image KAUST-7 was first investigated for SO 2 sorption, which is also one of the best physisorbent materials for capturing CO 2 at atmospheric concentration [44] with good water stability [45] . 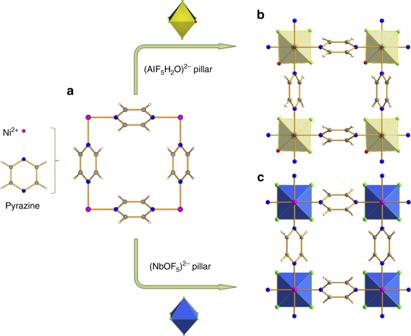Fig. 1 Synthesis and crystal structure of KAUST-7 and KAUST-8.a[Ni(pyrazine)2]2+square grid resulting from the connection of Ni2+cations and pyrazine molecules.bCrystal structure of KAUST-8 resulting from the pillaring of [Ni(pyrazine)2]2+square grid with (AlF5(OH2))2−pillar.cCrystal structure of KAUST-7 resulting from the pillaring of [Ni(pyrazine)2]2+square grid with (NbOF5)2−pillar The steep, pure SO 2 adsorption isotherm collected at 25 °C (Supplementary Figure 1 ) suggested a high affinity of the KAUST-7 framework for SO 2 . To gain better insight on the SO 2 position within the framework and the governing interactions responsible for resultant strong affinity, we performed in situ single crystal X-ray diffraction (SCXRD) study on a suitable single crystal of KAUST-7 at 296 K under 4–5 bar of SO 2 -containing atmosphere (7% SO 2 , 93% N 2 ). The structure analysis revealed that the resultant compound crystallized in the tetragonal space group P 4/ nbm with the unit cell parameters a = b = 9.9249(2) Å and c = 7.8387(2) Å (Supplementary Table 1 ). 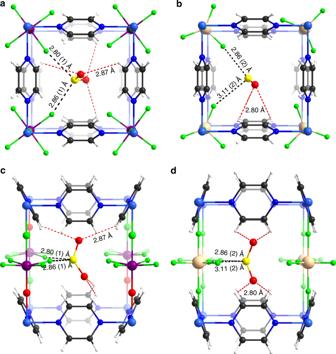Fig. 2 In situ visualization of SO2in host frameworks. Intermolecular host–guest interactions in SO2loaded crystal structures ofa,cKAUST-7 andb,dKAUST-8 An axial distortion of the octahedral (NbOF 5 ) 2− anion (Nb–O bond is shorter than Nb–F trans , 1.82(3) and 2.03(3) Å, respectively) was observed and manifested in a disorder in the structure: the Nb atom was split over two positions, whereas the oxygen and the trans -fluoride were refined in the same position with equal thermal parameters (Supplementary Figure 2a ). The fluorinated pillars are turned by φ = ±8.5(2)° from the direction toward the center of the channel (Supplementary Figure 2b ) depending on the central atom position. The (NbOF 5 ) 2− anion twist is stabilized by four pairs of C–H∙∙∙F hydrogen bonds with the adjacent pyrazine molecules: the H∙∙∙F distances and C–H∙∙∙F angles are 2.45 Å and 158° in the case of the Nb shifted toward that Ni(pyrazine) 2 layer, and 2.52 Å and 170° when in the opposite direction (Supplementary Figure 2 c and 2d ). The SO 2 molecule was localized in the center of the one-dimensional (1D) channel at a special position, similar to CO 2 molecule in the KAUST-7 (CO 2 )structure [44] . As the site symmetry (−42 m ) is higher than the symmetry of the guest molecule, the SO 2 is disordered over four positions around axis −4 with the total occupancy refined to 0.424(4). Contrary to the linear CO 2 molecule surrounded by four F-pillars, the electropositive sulfur atom of the triangular SO 2 molecule interacts with only two electronegative fluorine atoms of the adjacent (NbOF 5 ) 2− anions (S∙∙∙F distances of 2.80(1) and 2.86(1) Å) shown in Fig. 2a–c . In addition, the SO 2 molecule in the MOF is stabilized by four C–H∙∙∙O contacts with the hydrogen atoms of four different pyrazines (H∙∙∙O distance = 2.87 Å, angle = 120°). Fig. 2 In situ visualization of SO 2 in host frameworks. Intermolecular host–guest interactions in SO 2 loaded crystal structures of a , c KAUST-7 and b , d KAUST-8 Full size image This observation is corroborated by density functional theory (DFT) calculations, which revealed high SO 2 /KAUST-7 interaction energy of − 64.8 kJ mol −1 . 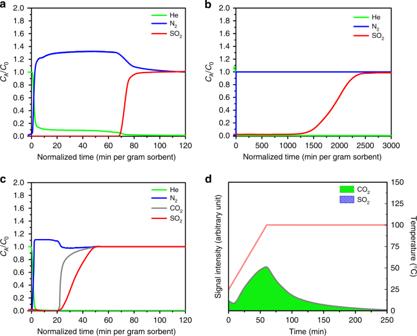Fig. 3 CO2/SO2capture performance of KAUST-7. Adsorption column breakthrough experiments for KAUST-7withaSO2/N2: 7/93 mixture (10 cm3min−1, flow rate),bSO2/N2: 0.05/99.95 mixture (40 cm3min−1, flow rate), andcSO2/CO2/N2: 0.05/10/89.95 mixture (25 cm3min−1, flow rate).dTemperature-programmed desorption after initial adsorption in the column using a mixture akin to flue gas (SO2/CO2/N2: 0.05/10/89.95), suggesting an adsorbed phase composition dominated by CO2 This is due to a relatively stronger interaction between the sulfur atom of SO 2 and the F-pillars with characteristic interatomic distances of 2.9 Å (Supplementary Figure 3a ) along with a charge transfer between the guest and this region of the MOF. Interestingly, the SO 2 /KAUST-7 interaction energy is as high as the value calculated for CO 2 (−54.5 kJ mol −1 ). This latter molecule occupies slightly different sites than SO 2 , implying an interaction of the guest molecule with both the F-pillars and the pyrazine groups (Supplementary Figure 3b ). The so-predicted energetics and spatial distributions for both molecules as single components suggest simultaneous capture of SO 2 and CO 2 . Cyclic adsorption column breakthrough tests with SO 2 /N 2 : 7/93 indicate stability and good uptake (≈2.2 mmol g −1 ) of SO 2 (Fig. 3a ). 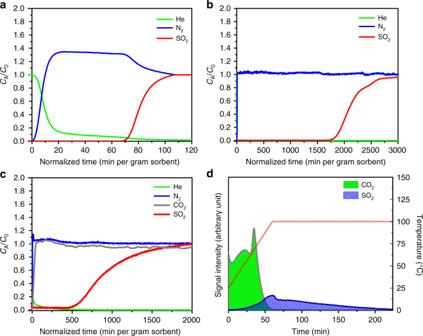Fig. 4 CO2/SO2capture performance of KAUST-8. Adsorption column breakthrough experiments for KAUST-8 withaSO2/N2: 7/93 (10 cm3min−1, flow rate),bSO2/N2: 0.05/99.95 mixture (40 cm3min−1, flow rate), andcSO2/CO2/N2: 0.05/10/89.95 (40 cm3min−1, flow rate).dTPD experiment suggests a considerable amount of SO2along with CO2as adsorbed phase after a breakthrough experiment with 500 p.p.m. SO2in the presence of 10% CO2and balance N2 Furthermore, adsorption column breakthrough experiments with SO 2 /CO 2 /N 2 : 4/4/92 gas mixture showed simultaneous and equal retention time in the column for SO 2 and CO 2 , demonstrating identical uptake of ≈1.1 mmol g −1 (Supplementary Figure 4 ), which is consistent with the simulated energetics trends. Upon decreasing the SO 2 concentration with nitrogen in the range commonly observed in flue gas (500 p.p.m.) (SO 2 /N 2 : 0.05/99.95 mixture) and the immediately dangerous to life or health concentration (100 p.p.m. ), KAUST-7 still maintains a high SO 2 uptake of about 1.4 mmol g −1 at 500 p.p.m. SO 2 concentration (Fig. 3b ). Interestingly, adsorption column breakthrough experiments under mimicked flue gas conditions with 500 p.p.m. of SO 2 and 10% CO 2 in N 2 (SO 2 /CO 2 /N 2 : 0.05/10/89.95) resulted in equal and simultaneous retention time for both SO 2 and CO 2 , leading to uptakes of ≈0.01 mmol g −1 and ≈2.2 mmol g −1 , respectively (Fig. 3c ). The direct co-adsorption experiments with different SO 2 and CO 2 compositions (4% SO 2 , 4% CO 2 , balance N 2 and 500 p.p.m. SO 2 , 10% CO 2 , balance N 2 ) demonstrate that KAUST-7 exhibits equal selectivity toward SO 2 and CO 2 (SO 2 /CO 2 selectivity ≈1), which is desirable for simultaneous CO 2 and SO 2 capture in flue gas (containing low SO 2 concentrations). Nevertheless, temperature-programmed desorption (TPD) confirmed the presence of CO 2 only with an undetectable amount of SO 2 (Fig. 3d ) in the adsorbed phase as the amount of SO 2 adsorbed is negligible owing to its low concentration. The performance of KAUST -7 using humid (≈40% Relative Humidity (RH)) 250 p.p.m. 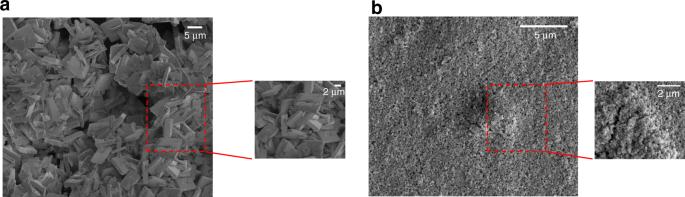Fig. 5 Scanning electron microscopy of thin films. SEM micrographs at a high and low magnification ofaKAUST-7 andbKAUST-8 thin films coated on the gold electrode of QCM SO 2 /balance N 2 gas mixture was also investigated (Supplementary Figure 5 ); it is evident that SO 2 has same breakthrough time as that of water and results in a lower SO 2 uptake under humid condition compared with the dry condition, which is not surprising considering the concentration of water is around 50 times higher than that of SO 2 . 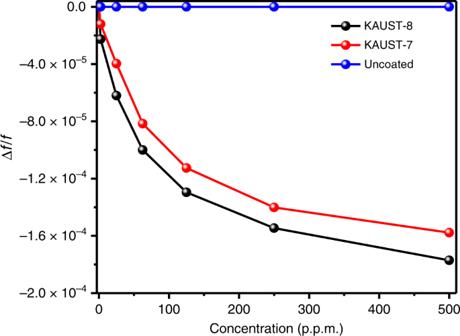Fig. 6 Frequency shift comparisons. Frequency shift as a function of the SO2concentration for the uncoated and KAUST-7- or KAUST-8-coated QCM sensors 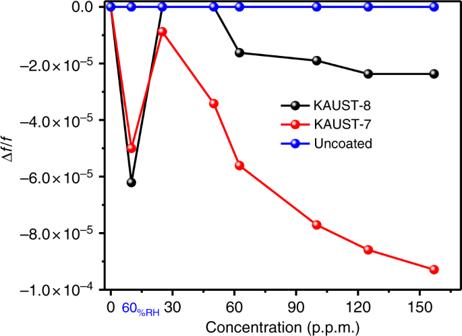Fig. 7 Sensor responses. Plots of sensors responses as a function of SO2concentration in synthetic air 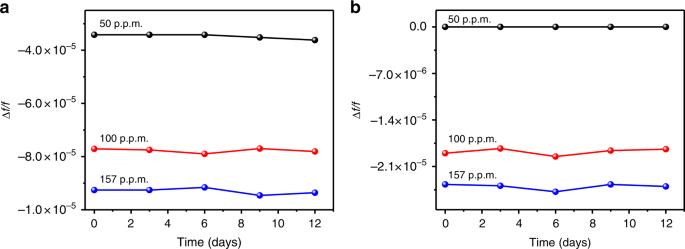Fig. 8 Stability and reproducibility. Long-term stability property of theaKAUST-7 andbKAUST-8 sensors exposed to 50, 100, and 157 p.p.m. SO2gas In addition to previously reported excellent water stability [44] , [45] , SO 2 stability of the KAUST -7 was proven by powder X-ray diffraction (PXRD) comparison of the materials before and after dry and humid SO 2 exposure (Supplementary Figure 6 ), CO 2 breakthrough study before and after 7% SO 2 breakthrough experiments (Supplementary Figure 7 ), and CO 2 adsorption isotherm after the humid SO 2 breakthrough experiment (Supplementary Figure 8 ). Fig. 3 CO 2 /SO 2 capture performance of KAUST -7 . Adsorption column breakthrough experiments for KAUST -7 with a SO 2 /N 2 : 7/93 mixture (10 cm 3 min −1 , flow rate), b SO 2 /N 2 : 0.05/99.95 mixture (40 cm 3 min −1 , flow rate), and c SO 2 /CO 2 /N 2 : 0.05/10/89.95 mixture (25 cm 3 min −1 , flow rate). d Temperature-programmed desorption after initial adsorption in the column using a mixture akin to flue gas (SO 2 /CO 2 /N 2 : 0.05/10/89.95), suggesting an adsorbed phase composition dominated by CO 2 Full size image In our quest for a material with a more favorable selectivity for SO 2 removal from flue gas than CO 2 (at 500 p.p.m. of SO 2 ), we opted to investigate an analog of KAUST -7 with lower CO 2 interactions and potentially higher SO 2 interactions. Inspired by our results with KAUST - 8 for dehydration of gases [46] and simultaneous removal of H 2 S/CO 2 [47] , we found it compelling to explore the structural SO 2 /CO 2 co-adsorption property. KAUST-8 exhibits three pendant fluoride groups with slightly higher F…F distance (3.613 Å) and one potential open metal site, whereas KAUST-7 contains four pendants fluoride with smaller F…F distance (3.210(8) Å) and no open metal site. Such minute differences in structural features led us to realize equal selectivity for CO 2 and H 2 S over a wide range of concentrations and temperatures [47] . Encouraged by this structure–property tuning of H 2 S and CO 2 adsorption affinity using this MOF, we expected KAUST-8 to be more selective toward SO 2 than CO 2 . Similar to gain better insight of the KAUST-8 system, SCXRD data were collected on the SO 2 -loaded KAUST-8 crystal. The structure analysis revealed the resultant compound crystallized in the tetragonal space group P 4/ mmm with the unit cell parameters a = b = 6.9996(2) Å and c = 7.7033(2) Å (Fig. 2b–d , Supplementary Table 2 ). Contrary to KAUST-7, a rotational disorder of the (AlF 5 ) 2− is caused by trigonal bipyramidal shape of the anions located at the axis 4 among four 1D channels in the structure. When one fluorine atom of a pillar is directed perfectly to the channel center ( φ = 0°), in the two other adjacent channels Al–F bonds of the same anion are directed ± 24.1(4)° out the diagonal direction, and in the fourth channel there are no F-atoms from this pillar (Supplementary Figure 9a ). Therefore, the single average cage aperture is formed by fluorine atoms of three adjacent (AlF 5 ) 2− anions only. The pillar twist is stabilized by three pairs of C–H∙∙∙F hydrogen bonds between the pyrazine molecules and the fluorine atoms with H∙∙∙F distances and C–H∙∙∙F angles of 2.38 Å and 178°, 2.48 Å and 134°, and 2.17 Å and 161°, respectively (Supplementary Figure 9 b and 9c ). Similar to SO 2 -loaded KAUST-7 structure, the guest SO 2 molecule is disordered in the center of the 1D channel (the special position symmetry is 4/ mmm ) of the KAUST-8 MOF. The distances between electropositive sulfur atom of the SO 2 molecule and fluorine atoms of adjacent F-pillars equals 2.86(2), 3.11(2), or 3.25(1) Å depending on the (AlF 5 ) 2− orientation ( φ = 0° or ± 24.1(4)°, Supplementary Figure 9d ) and each of them is less than the sum of the S and F van der Waals radii (3.27 Å). Contrary to the KAUST-7 structure, the SO 2 molecule participates in four C–H∙∙∙O contacts with only two neighboring pyrazines (H∙∙∙O distance = 2.80 Å, angle = 105°). These observations were supported by DFT calculations and it revealed a lowering of the host/guest interaction energy of CO 2 for KAUST-8 compared with KAUST-7 (− 47.0 kJ mol −1 vs. − 54.5 kJ mol −1 ). In the case of KAUST-8, the trigonal bipyramidal-like Al 3+ environment does not allow for further optimal interactions between a carbon atom in CO 2 and four F-pillars (Supplementary figure 3d ), as seen in KAUST-7. DFT calculations were further performed starting with the SO 2 -loaded crystal structure model elucidated from SCD data. Interestingly, the simulated preferential location of SO 2 is slightly pushed toward the pore wall, as compared with the scenario in KAUST-7, with the formation of a dual interaction between its sulfur atoms and the two nearby F-pillars, as well as its oxygen atoms interacting with the pyrazine linker with shorter interacting distances (Supplementary Figure 3c ). The resulting geometry led to a slight enhancement of the SO 2 /host interaction energy (− 73.9 kJ mol −1 ) and reduced affinity toward CO 2 , making KAUST-8 a promising candidate to selectively adsorb SO 2 over CO 2 . Investigation of single component SO 2 adsorption showed that KAUST-8 also exhibits steep adsorption isotherm at 25 °C (Supplementary Figure 10 ). The corresponding adsorption column breakthrough experiment with SO 2 /N 2 : 7/93 mixture showed a higher uptake of 2.2 mmol g −1 (Fig. 4a ). KAUST-8 can be completely regenerated by heating at 105 °C in a vacuum or inert gas environment (Supplementary Figure 11 ), confirming SO 2 stability and recyclability. During the adsorption column breakthrough experiments carried out with low SO 2 (SO 2 /N 2 : 0.05/99.95) mixture, KAUST-8 still maintained a high uptake of SO 2 (1.6 mmol g −1 ) (Fig. 4b , Supplementary Table 3 ). Subsequent TPD analysis of the adsorbed phase confirmed the adsorption of SO 2 (Supplementary Figure 12 ) at p.p.m. level. Supplementary Table 3 compares SO 2 uptake of different benchmark MOFs at low concentration. Materials with relatively more open structure such as MFM-300(In, Al) have very high SO 2 uptake at higher SO 2 concentration; however, they have lower SO 2 uptake at lower concentrations close to 500 p.p.m. (of interest for application such as SO 2 capture from flue gas and SO 2 sensing) compared with KAUST-7, KAUST-8, and some SIF 6 2− based MOFs. Materials such as MFM-300(In, Al) with very high SO 2 uptake at higher SO 2 concentration could have many important applications. MFM-300(In, Al) (very high uptake at higher concentration), and KAUST-7 and KAUST-8 (high uptake at very low concentration) are complementary to each other and their uses depend upon nature of the application. Adsorption column breakthrough experiments with synthetic flue gas using a SO 2 /CO 2 /N 2 : 0.05/10/89.95 mixture showed that SO 2 continues to be adsorbed for long durations past the CO 2 breakthrough time (Fig. 4c ). This indicates that the adsorbed CO 2 is replaced by SO 2 from the gas mixture, which is consistent with a much higher estimated interaction energy of SO 2 over CO 2 . Subsequent TPD analysis suggests an adsorbed phase composition of 1.5 mmol g −1 for CO 2 and 0.5 mmol g −1 for SO 2 , which is remarkable considering the large difference in concentrations of CO 2 and SO 2 in the synthetic flue gas (Fig. 4d ). A selectivity of SO 2 /CO 2 ≈ 66 obtained from the combination of breakthrough and TPD experiment shows that KAUST-8 is a highly efficient material for SO 2 removal at a p.p.m. level and is promising for selectively removing SO 2 from flue gas. The performance of KAUST-8 using humid (≈40% RH) 250 p.p.m. SO 2 / balance N 2 gas mixture was also investigated (Supplementary Figure 13 ). For KAUST-8, also SO 2 has almost the same breakthrough time as that of water; however, owing to its higher water adsorbing capacity than KAUST-7, it can adsorb more SO 2 compared with KAUST-7 under the same conditions. Uptake of SO 2 by KAUST-8 in humid condition is notable considering in the above experiment gas stream contained almost 50 times higher concentration of water than SO 2 . In addition to previously reported excellent water stability [46] , SO 2 stability of the KAUST-8 was proven by PXRD comparison of the materials before and after dry and humid SO 2 exposure (Supplementary Figure 14 ), CO 2 breakthrough study before and after 7% SO 2 breakthrough experiments (Supplementary Figure 15 ) and CO 2 adsorption isotherm after the humid SO 2 breakthrough experiment (Supplementary Figure 16 ). Fig. 4 CO 2 /SO 2 capture performance of KAUST - 8. Adsorption column breakthrough experiments for KAUST - 8 with a SO 2 /N 2 : 7/93 (10 cm 3 min −1 , flow rate), b SO 2 /N 2 : 0.05/99.95 mixture (40 cm 3 min −1 , flow rate), and c SO 2 /CO 2 /N 2 : 0.05/10/89.95 (40 cm 3 min −1 , flow rate). d TPD experiment suggests a considerable amount of SO 2 along with CO 2 as adsorbed phase after a breakthrough experiment with 500 p.p.m. SO 2 in the presence of 10% CO 2 and balance N 2 Full size image Selective SO 2 detection from air From the adsorptive separation study above, KAUST-8 and KAUST-7 were shown to exhibit tunable CO 2 /H 2 S selectivity, molecules that are present in environments contaminated with SO 2 . To benefit from the outstanding properties of this platform, we found it compelling to explore the feasibility of depositing KAUST-8 and KAUST-7 on a QCM electrode and unveiling their SO 2 sensing properties in the presence and absence of humidity to mimic atmospheric conditions. Weight-detectable sensor such as QCM has been used in this study to detect SO 2 accurately when the disturbing presence of moisture is involved. These imply that QCM device can be an alternative to IDE [48] when testing for a gas in the presence of humidity. Part of the reason for this difference is that IDE sensors are based on the change in dielectric constant ( ε H2O = 80 and ε SO2 = 16) and in order to detect SO 2 accurately in the presence of moisture the deposited materials on the IDE-type electrode has to overcome the high dielectric constant for H 2 O. The surface morphology of KAUST-8 and KAUST-7 coated on QCM (see inset) was studied using scanning electron microscopy. The thin films of both MOFs were found to be compact and uniform. The densely packed MOFs crystals were uniformly deposited on the QCM substrate with low intergranular voids and random orientation. As illustrated in Fig. 5 , the coating of KAUST-7 led to cubic crystallites of ~150 nm, whereas for the KAUST-8 films the size of the crystallites is significantly larger at ∼ 30 μm. PXRD experiments were carried out to confirm the purity and crystallinity of the deposited MOFs (Supplementary Figure 17 ). Fig. 5 Scanning electron microscopy of thin films. SEM micrographs at a high and low magnification of a KAUST-7 and b KAUST-8 thin films coated on the gold electrode of QCM Full size image The sensitivity (∆ f / f )) of KAUST-8- and KAUST-7-coated QCM devices were measured for different concentrations of SO 2 , ranging from 0 to 500 p.p.m. in balance with nitrogen [18] . Uncoated QCM showed a negligible response to SO 2 . With the increase in the concentration of SO 2 , both MOF-coated sensors responded with a nonlinear decrease in sensitivity (Fig. 6 ) and (Supplementary Figure 18 ). The lowest detection limit, defined theoretically using a largely accepted methodology by the sensing community [42] , was estimated to be about 100 p.p.b. (with noise drift in the resonance frequency of ± 1.5 Hz) [49] . By optimizing the device parameters, drift in the sensors resonance frequency, this detection limit can be reduced to below 0.2 Hz [50] , [51] and thereby improving the detection limit to < 15 p.p.b. This discrepancy/gap between the theoretical and experimental detection limits (15 p.p.b. and 5 p.p.m.) was never discussed previously in the open literature. Fig. 6 Frequency shift comparisons. Frequency shift as a function of the SO 2 concentration for the uncoated and KAUST-7- or KAUST-8-coated QCM sensors Full size image After each exposure cycle, the device was in situ heated at 105 °C in ambient nitrogen for 4 h, allowing the reactivation of the evaluated MOF thin film for another sensing cycle. Humidity is present in most environments, and so it is important to understand a sensors response in its presence. Therefore, mixed gas experiments were performed, exposing KAUST-7 and KAUST-8 to SO 2 in humid conditions mimicking real-world conditions for SO 2 detection. Figure 7 shows the sensor sensitivity as a function of SO 2 concentration in humid conditions (60% RH) at RT for uncoated and coated KAUST-7 and KAUST-8 QCMs. Uncoated QCM has a near-zero response to humidity and SO 2 . This corroborates that the sensing response to SO 2 under humid conditions is due to its affinity to KAUST-7 and KAUST-8 films. Fig. 7 Sensor responses. Plots of sensors responses as a function of SO 2 concentration in synthetic air Full size image The responses of the two kinds of sensors were different. As seen in Fig. 7 and (Supplementary Figure 19 ), the resonance frequency of the QCMs initially decreased when the ambience was changed from dry to humid SO 2 conditions. The most prominent difference is the inversion in the sensor output due to the introduction of SO 2 at 60% RH but not in the same manner as compared with the dry SO 2 case. Interestingly, when exposed to 25 p.p.m. of SO 2 in the above-mentioned humid conditions, the sensor resonance frequency for SO 2 was reduced. Under humid conditions, the sensitivity of the two MOFs slightly reduced when compared with dry conditions. However, KAUST-7 films demonstrated a four-time higher sensitivity toward SO 2 in the presence of humidity compared with KAUST-8. To further analyze the results obtained, it is necessary to consider the specific features of the adsorption of SO 2 and water on the surface of KAUST-7 and KAUST-8. As seen in Fig. 7 , the presence of humidity (60% RH) did not significantly affect the KAUST-7-based sensors response to the SO 2 analyte. This may be due to the affinity of SO 2 molecules to replace some of the adsorbed water molecules or/and coexist in the highly confined pore system. In the case of KAUST-8-based sensor, which is isomorphic to the KAUST-7, lower sensitivity to SO 2 in the presence of humidity was observed. Although SO 2 has the affinity to replace water molecules, the reduced sensitivity is attributed to the absence of accessible ultra-microporous morphology. The number of SO 2 -adsorbing active sites is reduced by the pre-adsorbed water, thereby limiting the available space in the pore system for adsorption. This observation is supported by the fact that the water molecules strongly interact with Al 3+ [46] with higher host/guest interaction energy as compared with SO 2 . The TPD experiment results (Supplementary Figure 20 ) show that in the case of KAUST-7, the SO 2 can replace the already adsorbed water molecules relatively easy as compared with the KAUST-8, which has stronger water affinity. These results are in agreement with the conclusion reported in the literature for the simultaneous capture of CO 2 and H 2 O using KAUST-8 [46] . The most important parameters for a sensing device are its stability and reproducibility. These parameters were investigated by cyclic exposure of the sensor to different SO 2 concentrations after every 48 h at RT over a period of 12 days (Fig. 8 ). The three results demonstrated the stability of the sensors exposed to 50, 100, and 157 p.p.m. SO 2 gas with no significant change in the resonant frequency over time. Fig. 8 Stability and reproducibility. Long-term stability property of the a KAUST-7 and b KAUST-8 sensors exposed to 50, 100, and 157 p.p.m. SO 2 gas Full size image In this report, we successfully demonstrated the superior performance of two fluorinated MOFs, namely KAUST-7 and KAUST-8, for the capture of SO 2 from flue gas. Combined mixed gas breakthrough experiments and molecular simulation confirmed that simultaneous capture of SO 2 and CO 2 occurs using KAUST-7, whereas KAUST-8 displays a higher affinity for SO 2 with SO 2 /CO 2 selectivity ≈66. Based on this performance, QCM-based sensors were successfully fabricated for sensing SO 2 from air using this fluorinated MOF platform (Supplementary Figure 21 ). Both MOF materials confirmed their potential, revealing good SO 2 detection capabilities above 25 p.p.m., the range of SO 2 concentrations in the air-inducing nose and eye irritation. This remarkable performance of sensing makes these materials highly desirable for the fabrication of new advanced devices to improve health and environmental conditions. Materials All reagents were used as received from commercial suppliers without further purification. KAUST-7 [44] , [45] and KAUST-8 [46] were synthesized according to literature procedures. Powder X-ray diffraction The PXRD data were collected over the 2 θ range 4–40° or 6–80° on a high-resolution PANalytical X’Pert MPD-PRO diffractometer with Cu K α 1 radiation ( λ = 1.5406 Å, 45 kV/40 mA). Single crystal X-ray diffraction The SCXRD data were collected using a Bruker X8 PROSPECTOR APEX2 CCD diffractometer (Cu K α, λ = 1.54178 Å). Indexings were performed using APEX2 (Difference Vectors method) [52] . Data integration and reduction were performed using SaintPlus [53] . Absorption corrections were performed by multi-scan method implemented in SADABS [54] . Space groups were determined using XPREP implemented in APEX2 [52] . Both structures were solved using Direct Methods (SHELXS-97) and refined using SHELXL-2018/3 (full-matrix least-squares on F 2 ) contained WinGX v1.70.01 [55] , [56] , [57] . In situ gas loading experiment We used commercially available Swagelok miniature quick connect with a small modification that allowed us to fix 0.3 mm glass capillary loaded with crystal above the quick connect. The selected single crystal was glued to glass fiber and placed in 0.3 mm glass capillary before attaching it to quick connect. In situ pretreatment of the crystal loaded in environmental gas cell was carried out first under dry nitrogen flow. Temperature of the crystal increased by immersing the capillary in to oil bath. Temperature of the oil bath was fixed at 140 °C for both the samples to obtain 105–120 °C effective temperature at the crystal. After 24 h, nitrogen flow was changed to dynamic vacuum keeping the temperature constant. After 12 h, crystal was allowed to cool down under dynamic vacuum and then 7% SO 2 (93% N 2 ) was introduced into environmental cell at 4–5 bar pressure. In case of CO 2 , 100% CO 2 was introduced at 2–3 bar. The gas-loaded environmental cell was detached under pressure and allowed to equilibrate for around 8 h. After 8 h, the environmental cell was mounted on a modified goniometer for single crystal X-ray data collection. Column breakthrough test set-up, procedure, and measurements The experimental setup used for dynamic breakthrough measurements is shown in Supplementary Figure 22 . The gas manifold consisted of three lines fitted with mass flow controllers. Line A is used to feed an inert gas, most commonly helium, to activate the sample before each experiment. The other two lines B and C feed a pure or pre-mixed gases. Whenever required, gases flowing through lines B and C may be mixed before entering a column packed with the sample using a four-way valve. In a typical experiment, 300–500 mg of adsorbent (in the column) was treated in situ at a required temperature under He flow (50 cm 3 g −1 ) for 8 h. Before starting each experiment, helium reference gas is flushed through the column and then the gas flow is switched to the desired gas mixture at the same flow rate between10–50 cm 3 g −1 . The gas mixture downstream the column was monitored using a Hiden mass spectrometer. Fabrication of KAUST-7- and KAUST-8-coated QCM The transducer was a 10 MHz AT-cut piezoelectric QCM device with a thickness shear mode and placed between two gold electrodes for electrical connection. The QCM is rinsed with ethanol and dried in air. MOFs paste was then applied to the electrode of QCMs by spin-coating method (2 μm thick); no prior modification of the sensors surface was required. The QCM sensor was then fixed in a sealed chamber. Before measurements, the fresh coated MOFs film was activated in situ for 4 h to have a guest free framework. The resulting coatings are ultrathin and reproducible so that the stress upon absorption of SO 2 inducing a change in the mass change of the thin film is effective. Sensing apparatus Supplementary Figure 23 shows the sensing setup used in this study for real-time measurement. All the sensor measurements were carried out at RT, under a dry air total stream of 200 cm 3 m −1 . MFCs (mass flow controllers) from Alicat Scientific, Inc. were used to control the flow rate for gases coming from certified bottles. Stainless steel delivery lines or perfluoroalkoxy alkane, Perfluoroalkoxy (PFA) tubing (in regions requiring flexibility and resistivity to volatile organic compounds (VOCs)) were used on the setup with Vernier metering valves (from Swagelok) as a flow regulator. To detect the change in humidity level inside the chamber, a commercial humidity sensor (Honeywell HIH-4000–003) was used as a reference, which has an error < 0.5% RH. The QCM sensor was exposed to the analyte stream until a stable response was obtained; a two-port network (Keysight E5071C ENA) circuit was used to monitor the change in resonance frequency. A LabVIEW interface was used for synchronization and data acquisition by controlling the LCR meter (L = Inductance, C = Capacitance, R = Resistance) and the multimeter. Hence, the possibility of data loss was minimized. Computational methods All simulations were performed using the codes available in the Quantum Espresso package [58] , which implements the DFT under periodic boundary conditions with planewave functions as basis sets [59] . The geometry optimizations were performed with the generalized gradient approximation (Perdew-Burke-Ernzerhof (PBE)) [60] including the dispersion corrections described by the Grimme’s scheme [61] , maintaining fixed the atomic coordinates of the F-Ni-F chains and the unit cell dimensions. The relative ion positions were relaxed until all of the force components were lower than 0.001 Ry Bohr −1 . The equilibrium atomic positions of all systems were found by minimizing the total energy gradient. The ion cores were described by Vanderbilt ultrasoft pseudopotential [62] and the Kohn–Sham one-electron states were expanded in a planewave basis set with a kinetic cutoff energy of 50 Ry (500 Ry for the density) All the calculations were performed at the Γ-point. The Hubbard approach was also applied in order to better describe the localized d states of nickel. The Hubbard parameters ( U ) were taken from the calculations of Wang et al. [63] , with a value of 6.4 eV for nickel. The Marzari–Vanderbilt smearing technique was used [64] with a broadening of 0.005 Ry in order to smooth the Fermi distribution. The geometry optimizations of SO 2 and CO 2 in both MOFs were performed by considering one guest molecule per formula unit. The interaction energy was then calculated using the following equation: Δ E = E MOF/guest molecule − E guest molecule − E empty MOF , where E MOF/guest molecule , E guest molecule , and E empty MOF are the total energy of the loaded system (guest molecule + MOF), of the guest molecule and the single-point total energy of the MOF, respectively.